Differential affinity of FLIP and procaspase 8 for FADD’s DED binding surfaces regulates DISC assembly Death receptor activation triggers recruitment of FADD, which via its death effector domain (DED) engages the DEDs of procaspase 8 and its inhibitor FLIP to form death-inducing signalling complexes (DISCs). The DEDs of FADD, FLIP and procaspase 8 interact with one another using two binding surfaces defined by α1/α4 and α2/α5 helices, respectively. Here we report that FLIP has preferential affinity for the α1/α4 surface of FADD, whereas procaspase 8 has preferential affinity for FADD’s α2/α5 surface. These relative affinities contribute to FLIP being recruited to the DISC at comparable levels to procaspase 8 despite lower cellular expression. Additional studies, including assessment of DISC stoichiometry and functional assays, suggest that following death receptor recruitment, the FADD DED preferentially engages FLIP using its α1/α4 surface and procaspase 8 using its α2/α5 surface; these tripartite intermediates then interact via the α1/α4 surface of FLIP DED1 and the α2/α5 surface of procaspase 8 DED2. Programmed cell death (apoptosis) plays a key role in maintaining normal tissue homoeostasis [1] . Dysfunctional apoptosis can result in autoimmune and neurodegenerative diseases and cancer [2] , [3] , [4] . Apoptosis is orchestrated by the caspase family of cysteine proteases whose activation is tightly controlled [5] . Activation of initiator caspases is achieved through adaptor-induced oligomerization and formation of multi-protein complexes [6] , [7] . The complex formed following activation of the CD95 (Fas) and DR4/DR5 death receptors is called the death-inducing signalling complex (DISC), which consists of the receptors, the adaptor molecule FADD (Fas-Associated Death Domain), procaspase 8, (FADD-like interleukin-1β-converting enzyme (FLICE)) and its inhibitor FLIP (FLICE-like inhibitory protein) [8] , [9] , [10] , [11] . FADD is recruited to the DISC by homotypic interactions between its death domains (DD) and the intracellular DD of Fas, DR4 or DR5 (ref. 12 ). FADD also regulates cell death signalling from TNFR1 Complex II and the Ripoptosome [13] , [14] . Interaction with death receptors exposes the FADD N-terminal death effector domain (DED), which recruits procaspase 8 by interacting with its N-terminal tandem DEDs [15] . Procaspase 8 dimerization results in conformational changes in its catalytic domains that lead to its activation and initiation of a proteolytic apoptotic cascade [16] . Procaspase 10 also contains tandem DEDs and can be recruited to the DISC, although its ability to compensate for the loss of procaspase 8 is controversial [10] , [17] , [18] . Three splice forms of FLIP have been identified: a long form (FLIP(L)) and two short forms (FLIP(S) and FLIP(R)), all of which contain tandem DEDs that can bind to FADD [19] , [20] . The ratio of FLIP to procaspase 8 molecules at the DISC is a key determinant of cell fate as FLIP can compete with procaspase 8 for DISC recruitment, preventing its activation [21] . In recent years, several structural and biochemical studies have shed new light on DISC assembly, and a new picture of this multi-protein signalling complex is emerging [22] , [23] , [24] , [25] , [26] . In this study, we have combined molecular modelling, functional assays and quantitative DISC analyses to identify the favoured modes of interaction and stoichiometry of the DEDs of FADD, FLIP and procaspase 8 at the DR5 DISC. Our findings suggest a mechanism of DISC assembly at the level of these DED-containing proteins and reveal important differences between FLIP and procaspase 8 in terms of their preferred modes of interaction with FADD that could be therapeutically exploited to promote apoptosis. DR5 DISC IP assay To assess FADD, FLIP and procaspase 8 recruitment to the DR5 DISC, we developed a DISC IP assay using a fully humanized DR5 agonistic antibody that binds the extracellular domain of DR5 (ref. 27 ) ( Supplementary Fig. 1A ); this DISC IP assay was validated using wild-type and FADD null Jurkat cell lines ( Supplementary Fig. 1B ). In parental Jurkat cells, FLIP(L) was present at the DISC exclusively in its caspase 8-processed p43-form, and FLIP(S), the less-abundant splice form in this cell line, was also recruited. Processing of DISC-recruited procaspase 8 was also evident. As expected, in FADD null Jurkats, crosslinked DR5 was unable to recruit FLIP or procaspase 8. Assessment of DISC stoichiometry To quantify the relative levels of FLIP, procaspase 8 and FADD recruited to the DR5 DISC, quantitative western blot analyses of DR5 DISC IP samples were performed using recombinant proteins for FLIP, FADD and caspase 8 as standards, analysed alongside DISC IP samples from A549, H460 and HCT116 cells ( Fig. 1a ). Standard curves for each recombinant protein were generated ( Fig. 1b ), and from these, the amounts of FLIP, FADD and caspase 8 present at the DR5 DISCs formed in each cell line were calculated ( Fig. 1c ). Subsequently, the ratios of the three proteins to one another were calculated for each cell line model; the average ratios from three independent experiments are shown in Fig. 1d . As expected, in the most TRAIL-resistant cell line, A549, the ratio of FLIP to FADD and FLIP to caspase 8 was highest, whereas the TRAIL-sensitive HCT116 and H460 cells had lower FLIP:FADD and FLIP:caspase 8 ratios. These TRAIL-sensitive models also had higher caspase 8:FADD ratios than the A549 cell line. Notably, for every FADD molecule recruited, there were approximately two FLIP/procaspase 8 molecules recruited. We also performed time-course experiments in the A549 cell line, which showed that the ratio of FLIP to caspase 8 and FADD remained relatively constant over time ( Fig. 1e ). When the DISC IP was repeated in A549 cells with lower amounts of DR5 agonistic antibody, the ratio of FLIP to FADD and FLIP to caspase 8 were both close to one ( Fig. 1f ); this suggests that for low levels of DR5 activation, there is a 1:1:1 ratio of the DED proteins at the DISC. In addition, quantitative western blotting was used to estimate the number of FLIP, FADD and procaspase 8 molecules in A549 and H460 cells; FLIP was expressed ~20 and ~50 times lower than procaspase 8 and ~20 and ~25 times lower than FADD in A549 and H460 cells respectively; these ratios again correlated with the relative TRAIL sensitivity of these cell lines. 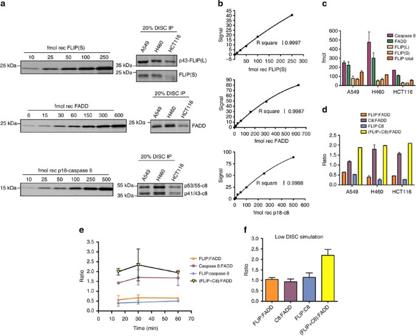Figure 1: Assessment of DR5 DISC stoichiometry. (a) Quantitative western blot analysis of FLIP, FADD and caspase 8 levels in DR5 DISC IP samples was carried out in A549, H460 and HCT116 cells seeded at 5 × 106and exposed the next day to equal amounts of the agonistic anti-DR5 antibody crosslinked to magnetic beads for 30 min. For each protein, 20% of the DISC IP sample was assessed alongside serial dilutions of each recombinant protein: His-tagged FLIP(S); untagged FADD and p18-caspase 8. (b) Bands were detected and quantified using the Odyssey Infrared Imaging System (LI-COR Biosciences). Standard curves were generated for each recombinant protein. These were second-order polynomials, from which the absolute amounts of FLIP, FADD and caspase 8 recruited to the DISC were calculated. (c) Femtomoles (fmol) of FLIP, FADD and caspase 8 recruited to the DR5 DISC in A549, H460 and HCT116 cells. For caspase 8, the levels of p53/55 and p41/p43-caspase 8 were added together. For FLIP, p43-FLIP(L) and FLIP(S) were added together. The result of a representative experiment is presented. (d) Ratios of the fmol of FLIP to FADD and caspase 8, caspase 8 to FADD and FLIP/caspase 8 to FADD recruited to the DR5 DISC in A549, H460 and HCT116 cells. The mean ratios and s.d. from three independent experiments are shown. (e) Ratios of the amount of FLIP to FADD and caspase 8, caspase 8 to FADD and FLIP/caspase 8 to FADD recruited to the DR5 DISC in A549 cells treated for 15, 30 and 60 min with anti-DR5-conjugated magnetic beads. The mean ratios and s.d. from three independent experiments are shown. (f) The ratios of DED-containing proteins to one another were calculated from DR5 DISC IP experiments using sub-lethal amounts of anti-DR5-conjugated magnetic beads. In these experiments, A549 cells were treated with 25% the number of beads used in other experiments. The mean ratios and standard deviations from three independent experiments are shown. Figure 1: Assessment of DR5 DISC stoichiometry. ( a ) Quantitative western blot analysis of FLIP, FADD and caspase 8 levels in DR5 DISC IP samples was carried out in A549, H460 and HCT116 cells seeded at 5 × 10 6 and exposed the next day to equal amounts of the agonistic anti-DR5 antibody crosslinked to magnetic beads for 30 min. For each protein, 20% of the DISC IP sample was assessed alongside serial dilutions of each recombinant protein: His-tagged FLIP(S); untagged FADD and p18-caspase 8. ( b ) Bands were detected and quantified using the Odyssey Infrared Imaging System (LI-COR Biosciences). Standard curves were generated for each recombinant protein. These were second-order polynomials, from which the absolute amounts of FLIP, FADD and caspase 8 recruited to the DISC were calculated. ( c ) Femtomoles (fmol) of FLIP, FADD and caspase 8 recruited to the DR5 DISC in A549, H460 and HCT116 cells. For caspase 8, the levels of p53/55 and p41/p43-caspase 8 were added together. For FLIP, p43-FLIP(L) and FLIP(S) were added together. The result of a representative experiment is presented. ( d ) Ratios of the fmol of FLIP to FADD and caspase 8, caspase 8 to FADD and FLIP/caspase 8 to FADD recruited to the DR5 DISC in A549, H460 and HCT116 cells. The mean ratios and s.d. from three independent experiments are shown. ( e ) Ratios of the amount of FLIP to FADD and caspase 8, caspase 8 to FADD and FLIP/caspase 8 to FADD recruited to the DR5 DISC in A549 cells treated for 15, 30 and 60 min with anti-DR5-conjugated magnetic beads. The mean ratios and s.d. from three independent experiments are shown. ( f ) The ratios of DED-containing proteins to one another were calculated from DR5 DISC IP experiments using sub-lethal amounts of anti-DR5-conjugated magnetic beads. In these experiments, A549 cells were treated with 25% the number of beads used in other experiments. The mean ratios and standard deviations from three independent experiments are shown. Full size image Two potential orientations for the FLIP–FADD interaction To investigate the molecular basis for FLIP’s ability to compete with procaspase 8 for DISC binding despite its apparent lower expression, we employed computational techniques to study the interaction between FLIP and FADD. A homology model of human FLIP DED1 and DED2 based on the X-ray structure of viral FLIP MC159 ( PDB id 2BBR ) was constructed ( Fig. 2a ). This model indicated that the DED1/DED2 intra-molecular interface involved interactions between F23 of DED1 α2 and hydrophobic residues of DED2, which form a hydrophobic groove between α1 and α4 ( Fig. 2b ). On the DED2 surface, A98 is positioned between α2 and α5 of DED1. F23 belongs to the hydrophobic patch of DED1 and is highly conserved among DED-containing proteins; the corresponding residues on DED2 and DED surfaces of FLIP and FADD are F114 and F25 respectively, while in procaspase 8, they are F24 and F122 in DED1 and DED2, respectively ( Supplementary Fig. 2A ). A98 is also conserved in its hydrophobic nature; however, in FLIP DED1, FADD DED and procaspase 8 DED1 and DED2 it is either histidine or tyrosine. The conserved nature of the DEDs allowed us to develop a shorthand way of depicting them as chevrons ( Supplementary Fig. 2B ). 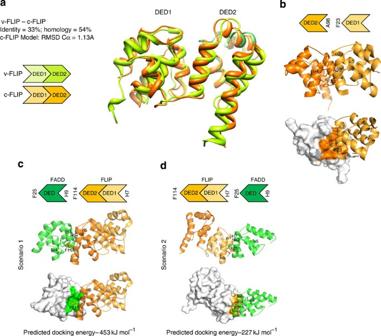Figure 2: Molecular modelling identifies two potential orientations for the FLIP–FADD interaction. (a) Homology model of human FLIP DED1 and DED2 (light and dark orange) superimposed on vFLIP X-ray protein (PDB id 2BBR; light green and green) and α3 region of FADD NMR-solved structure (PDB id 2GF5; dark green). The two DEDs (light and dark colours) are symmetrical and they are each composed of six α-helices. The human FLIP MC159 identity is 33%; the r.m.s.d. calculated on Cα atoms is 1.16 Å. (b) DED1/DED2 interactions within human FLIP. Hydrophobic interactions are centred on F23 located on α2 of DED1, which is accommodated into a hydrophobic groove between α1 and α4 of DED2. Two surfaces (α1/α4 and α2/α5) are involved in the intra- and intermolecular homotypic interactions between DEDs. On these surfaces, conserved hydrophobic residues are responsible for DED interactions: F on α2/α5 surface and (A)H/Y residues on α1/α4. Two possible orientations of FLIP/FADD interaction and their predicted docking energies are depicted: (c) F114 located on α2 helix of FLIP DED2 is accommodated into a hydrophobic groove formed between α1 and α4 helices of FADD DED; (d) F25 located on α2 helix of FADD DED is accommodated into an hydrophobic groove formed between α1 and α4 helices of FLIP DED1. Figure 2: Molecular modelling identifies two potential orientations for the FLIP–FADD interaction. ( a ) Homology model of human FLIP DED1 and DED2 (light and dark orange) superimposed on vFLIP X-ray protein (PDB id 2BBR; light green and green) and α3 region of FADD NMR-solved structure (PDB id 2GF5; dark green). The two DEDs (light and dark colours) are symmetrical and they are each composed of six α-helices. The human FLIP MC159 identity is 33%; the r.m.s.d. calculated on Cα atoms is 1.16 Å. ( b ) DED1/DED2 interactions within human FLIP. Hydrophobic interactions are centred on F23 located on α2 of DED1, which is accommodated into a hydrophobic groove between α1 and α4 of DED2. Two surfaces (α1/α4 and α2/α5) are involved in the intra- and intermolecular homotypic interactions between DEDs. On these surfaces, conserved hydrophobic residues are responsible for DED interactions: F on α2/α5 surface and (A)H/Y residues on α1/α4. Two possible orientations of FLIP/FADD interaction and their predicted docking energies are depicted: ( c ) F114 located on α2 helix of FLIP DED2 is accommodated into a hydrophobic groove formed between α1 and α4 helices of FADD DED; ( d ) F25 located on α2 helix of FADD DED is accommodated into an hydrophobic groove formed between α1 and α4 helices of FLIP DED1. Full size image We hypothesized that FLIP–FADD inter-molecular interactions should follow similar principles to the DED1–DED2 intra-molecular interactions. Protein–protein docking between FLIP and FADD indicated two potential orientations for the FLIP–FADD interaction: FLIP F114 binding into the FADD α1/α4 groove with a reciprocal interaction from FADD H9 into the α2/α5 hydrophobic patch of FLIP DED2 ( Fig. 2c ), and FADD F25 binding into the α1/α4 groove of FLIP DED1 with a reciprocal interaction from FLIP H7 into the α2/α5 hydrophobic patch of FADD’s DED ( Fig. 2d ). Interestingly, the predicted docking energies for the two orientations were significantly different. Predominant orientation of the FLIP–FADD interaction To test the modelling predictions, we generated Flag-tagged F114A, H7G and F114A/H7G mutant FLIP(S) expression constructs and assessed the ability of the mutants to bind to the FADD DED in GST pull-down assays. Interaction of the F114A mutant, but not H7G, with rFADD was significantly attenuated ( Fig. 3a ). Similarly, binding of FLIP(L) to FADD was abrogated by mutation of F114, but not H7 ( Fig. 3b ). Strikingly, even swapping the phenyl of F114 to the phenol of tyrosine was sufficient to attenuate the interaction between FLIP and FADD ( Fig. 3c ), further indicating the importance of this residue. To confirm the predominant direction of the FLIP–FADD interaction, we generated FADD F25A, H9G and F25A/H9G mutants and performed a pull-down assay using wild-type GST-FLIP(S) as bait. In agreement with the above results, H9G, but not F25A, mutant FADD, interacted significantly less than the wild-type protein ( Fig. 3d ). Further analyses using wild-type GST-FLIP(S) as bait demonstrated that mutating H9 to alanine had the same effect as mutating it to glycine ( Fig. 3e ). 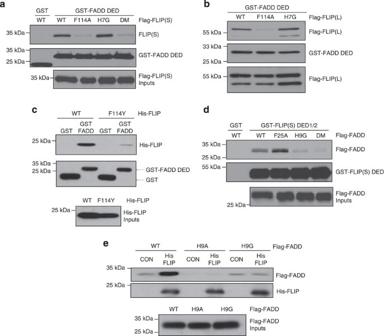Figure 3: Mutagenesis reveals the predominant orientation for the FLIP–FADD interaction. (a) Western blot analysis of GST pull-down assay using FADD DED as bait and wild-type and mutant human Flag-FLIP(S) as prey. (b) Western blot analysis of GST pull-down assay using FADD DED as bait and wild-type and mutant human Flag-FLIP(L) as prey. (c) Western blot analysis of GST pull-down assay using FADD DED as bait and His-tagged recombinant wild-type and F114Y mutant FLIP(S) as prey. (d) Western blot analysis of GST pull-down assay using FLIP(S) as bait and wild-type and mutant Flag-FADD as prey. (e) Western blot analysis of His pull-down assay using His-FLIP(S) as bait and wild-type and H9A and H9G mutant Flag-FADD as prey. Figure 3: Mutagenesis reveals the predominant orientation for the FLIP–FADD interaction. ( a ) Western blot analysis of GST pull-down assay using FADD DED as bait and wild-type and mutant human Flag-FLIP(S) as prey. ( b ) Western blot analysis of GST pull-down assay using FADD DED as bait and wild-type and mutant human Flag-FLIP(L) as prey. ( c ) Western blot analysis of GST pull-down assay using FADD DED as bait and His-tagged recombinant wild-type and F114Y mutant FLIP(S) as prey. ( d ) Western blot analysis of GST pull-down assay using FLIP(S) as bait and wild-type and mutant Flag-FADD as prey. ( e ) Western blot analysis of His pull-down assay using His-FLIP(S) as bait and wild-type and H9A and H9G mutant Flag-FADD as prey. Full size image We subsequently assessed the ability of wild-type and mutant FLIP(S) proteins to be recruited to the DR5 DISC and block TRAIL-induced apoptosis. Consistent with the results from the GST pull-down experiments, F114A mutant FLIP(S) also exhibited diminished recruitment to the DISC in HCT116 cells, whereas H7G FLIP(S) was recruited ( Fig. 4a ). Moreover, stable overexpression of wild-type but not F114A mutant FLIP(S) attenuated TRAIL-induced apoptosis ( Fig. 4b ), IETD-ase (caspase 8-like) and DEVD-ase (caspase 3/7-like) activity ( Fig. 4c ) in HCT116 colorectal cancer cells. In contrast, H7G mutant FLIP blocked TRAIL-induced caspase activation and apoptosis with a similar efficiency to the wild-type protein ( Fig. 4b,c ). These findings were confirmed in H460 non-small cell lung cancer cells, in which stably over-expressed wild-type and H7G mutant FLIP(S) were recruited to the DISC and blocked processing of caspase 8 to its p18-form ( Fig. 4d ), whereas the F114A mutant form was not recruited and failed to block TRAIL-induced caspase 8 processing. Mutation of F114 in FLIP(L) also attenuated its recruitment to the DR5 DISC ( Fig. 4e ), while mutation of additional amino acids on the α2/α5 surface of FLIP DED2 identified two further residues, K117 and K154, which are involved in FLIP’s DISC recruitment ( Fig. 4f ). In contrast, mutation of three residues (E4, E11 and E46) on the α1/α4 surface that molecular modelling suggested would be involved in mediating the alternative orientation of the interaction had no effect on FLIP’s DISC recruitment ( Fig. 4f ). 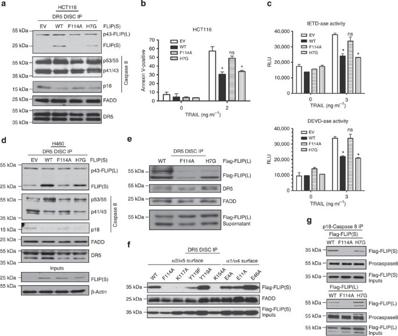Figure 4: Functional confirmation of the predominant orientation of the FLIP–FADD interaction. (a) Western blot analysis of DR5 DISC IP carried out in HCT116 cells stably over-expressing wild-type and mutant FLIP(S). The DR5 DISC was captured 1 h after addition of anti-DR5-conjugated beads to cells. Co-immunoprecipitation of FLIP, FADD and caspase 8 was assessed and pull down of DR5 confirmed. (b) Annexin V/propidium iodide flow cytometry analysis of apoptosis in control HCT116 cells (EV) and HCT116 cells stably expressing wild-type (WT) or F114A or H7G mutant FLIP(S). Cells were treated with 2 ng ml−1rTRAIL for 16 h; mean values and s.d. are shown (n=3). (c) Caspase 8-like (IETD-ase) and caspase 3/7-like (DEVD-ase) activity in control HCT116 cells (EV) and HCT116 cells stably expressing wild-type (WT) or F114A or H7G mutant FLIP(S). Cells were treated with indicated concentrations of rTRAIL for 16 h; mean values and s.d. are shown (n=3). (d) Western blot analysis of DR5 DISC IP carried out in H460 NSCLC cells stably over-expressing wild-type and mutant FLIP(S). The DR5 DISC was captured 1 h after addition of anti-DR5-conjugated beads to cells. Co-immunoprecipitation of FLIP, FADD and caspase 8 was assessed and pull down of DR5 confirmed. (e) Western blot analysis of DR5 DISC IP carried out in HCT116 cells transfected with wild-type and mutant Flag-FLIP(L) constructs. Cells were transfected for 24 h prior to treatment. The DR5 DISC was captured 1 h after addition of anti-DR5-conjugated beads to cells. Co-immunoprecipitation of Flag-tagged FLIP(L) and FADD was assessed and pull down of DR5 confirmed. (f) Western blot analysis of DR5 DISC IP carried out in HCT116 cells transfected with wild-type and mutant Flag-FLIP(S) constructs. The DR5 DISC was captured 1 h after addition of anti-DR5-conjugated magnetic beads to cells. Co-immunoprecipitation of Flag-tagged FLIP and endogenous FADD was assessed. (g) Western blot analysis of caspase 8 IP carried out in HCT116 colon cancer cells transfected with Flag-tagged wild-type or mutant FLIP(S) and FLIP(L) expression constructs. Twenty-four hours after transfection, cells were pre-treated with 10 μM z-VAD-fmk for 1 h prior to treatment with 5 ng ml−1rTRAIL for a further hour. Immunoprecipitates were analysed for the presence of Flag-tagged proteins. *; ns, non-significant compared with EV control as determined byt-test. Figure 4: Functional confirmation of the predominant orientation of the FLIP–FADD interaction. ( a ) Western blot analysis of DR5 DISC IP carried out in HCT116 cells stably over-expressing wild-type and mutant FLIP(S). The DR5 DISC was captured 1 h after addition of anti-DR5-conjugated beads to cells. Co-immunoprecipitation of FLIP, FADD and caspase 8 was assessed and pull down of DR5 confirmed. ( b ) Annexin V/propidium iodide flow cytometry analysis of apoptosis in control HCT116 cells (EV) and HCT116 cells stably expressing wild-type (WT) or F114A or H7G mutant FLIP(S). Cells were treated with 2 ng ml −1 rTRAIL for 16 h; mean values and s.d. are shown ( n =3). ( c ) Caspase 8-like (IETD-ase) and caspase 3/7-like (DEVD-ase) activity in control HCT116 cells (EV) and HCT116 cells stably expressing wild-type (WT) or F114A or H7G mutant FLIP(S). Cells were treated with indicated concentrations of rTRAIL for 16 h; mean values and s.d. are shown ( n =3). ( d ) Western blot analysis of DR5 DISC IP carried out in H460 NSCLC cells stably over-expressing wild-type and mutant FLIP(S). The DR5 DISC was captured 1 h after addition of anti-DR5-conjugated beads to cells. Co-immunoprecipitation of FLIP, FADD and caspase 8 was assessed and pull down of DR5 confirmed. ( e ) Western blot analysis of DR5 DISC IP carried out in HCT116 cells transfected with wild-type and mutant Flag-FLIP(L) constructs. Cells were transfected for 24 h prior to treatment. The DR5 DISC was captured 1 h after addition of anti-DR5-conjugated beads to cells. Co-immunoprecipitation of Flag-tagged FLIP(L) and FADD was assessed and pull down of DR5 confirmed. ( f ) Western blot analysis of DR5 DISC IP carried out in HCT116 cells transfected with wild-type and mutant Flag-FLIP(S) constructs. The DR5 DISC was captured 1 h after addition of anti-DR5-conjugated magnetic beads to cells. Co-immunoprecipitation of Flag-tagged FLIP and endogenous FADD was assessed. ( g ) Western blot analysis of caspase 8 IP carried out in HCT116 colon cancer cells transfected with Flag-tagged wild-type or mutant FLIP(S) and FLIP(L) expression constructs. Twenty-four hours after transfection, cells were pre-treated with 10 μM z-VAD-fmk for 1 h prior to treatment with 5 ng ml −1 rTRAIL for a further hour. Immunoprecipitates were analysed for the presence of Flag-tagged proteins. *; ns, non-significant compared with EV control as determined by t -test. Full size image To confirm the results of the DISC IP assay, we further investigated wild-type and mutant FLIP DISC recruitment by immunoprecipitating caspase 8 from TRAIL-treated cells using an antibody that recognizes its p18 subunit. In agreement with the results described above, binding of F114A mutant FLIP(S) and FLIP(L) to procaspase 8 was completely abrogated compared with wild-type FLIP in TRAIL-treated cells; however, binding of H7G mutant FLIP was similar to wild type ( Fig. 4g ). We recently reported that Ren mesothelioma cells are resistant to TRAIL, but are sensitized to TRAIL-induced apoptosis when FLIP expression is downregulated by siRNA or the histone deacetylase inhibitor, suberoylanilide hydroxamic acid (SAHA) [28] . We found that stable overexpression of wild-type and H7G mutant FLIP(S), but not the F114A mutant, blocked the synergistic interaction between TRAIL and SAHA or FLIP siRNA in Ren cells as assessed in cell viability analyses ( Supplementary Fig. 3A,B ). Collectively, the above experiments indicate that of the two possible orientations for the FLIP–FADD interaction, the orientation depicted in Fig. 2c is the predominant one during TRAIL-induced apoptosis, in agreement with the docking energies predicted for the two orientations. Furthermore, this also appears to hold true not only for the TRAIL DISC but also for TNFR1 Complex II, as H7G but not F114A mutant FLIP(S) blocked apoptosis induced by this complex ( Supplementary Fig. 3C ). The FLIP ‘charged triad’ is also essential for FADD binding Earlier studies using viral FLIP MC159 suggested that so-called ‘charged triad’ E/D-RxDL motifs present in its DEDs were important for its anti-apoptotic activity [29] , [30] ; these charged triad motifs are also present in cellular FLIP, FADD and DED1 of procaspase 8 (ref. 30 ) ( Supplementary Fig. 2A,B ). We generated Flag-tagged versions of human FLIP(S) with mutations in the charged triads of DED1 (R64A/D66A) and DED2 (R161A/D163A) and a double mutant (R64A/D66A/R161A/D163A). Unlike murine FLIP(R) [31] , human FLIP(S) required both the DED1 and DED2 charged triads in order to interact with FADD and be recruited to the DISC ( Supplementary Fig. 4A,B ). Modelling analyses revealed why the charged triad in FLIP DED2 is important: the E/D-RxDL motif acts as an ‘anchor’ that maintains the structural topography of the hydrophobic region formed by the α2 and α5 helices that engages H9 of FADD ( Supplementary Fig. 4C ). It is likely that the charged triad motif in FLIP DED1 is important for maintaining the ‘dumbbell’ structure of the tandem DEDs by orientating F23 into the hydrophobic groove between α1 and α4 ( Fig. 2b ). Predominant orientation of the procaspase 8–FADD interaction The results described above indicate that FLIP most efficiently binds to the α1/α4 surface of FADD, suggesting that procaspase 8 must engage this surface of FADD to initiate apoptosis. To assess this, we generated a homology model of procaspase 8 DED1 and DED2, again using viral FLIP MC159 as template ( Fig. 5a ). As previously observed in FLIP, the highly conserved F24 residue of procaspase 8 DED1 α2 is accommodated into a hydrophobic groove formed by DED2 α1/α4, while Y106 points into the hydrophobic patch of DED1 α2/α5. When protein–protein docking was assessed, two possible orientations for the interaction were again obtained, with either procaspase 8 F122 binding into the FADD α1/α4 groove with a reciprocal interaction from FADD H9 into the α2/α5 hydrophobic patch of procaspase 8 DED2 ( Fig. 5b ) or FADD F25 binding into the α1/α4 groove of procaspase 8 DED1 with a reciprocal interaction from procaspase 8 Y8 into the α2/α5 hydrophobic patch of FADD’s DED ( Fig. 5c ). 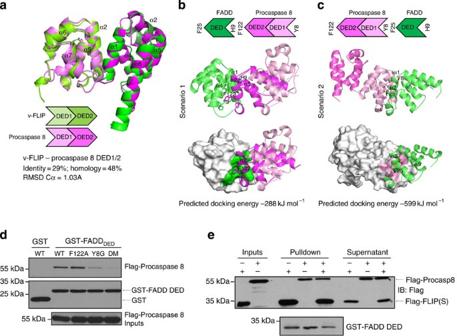Figure 5: Molecular modelling and mutagenesis identify the predominant orientation for the procaspase 8–FADD interaction. (a) Homology model of human procaspase 8 DED1 and DED2 (light and dark magenta) superimposed on vFLIP X-ray protein (PDB id 2BBR; light green and green) and α3 region of FADD NMR-solved structure (PDB id 2GF5; dark green). The procaspase 8 DED1/2-MC159 identity is 29%; the r.m.s.d. calculated on Cα atoms is 1.03 Å. Two possible orientations of the procaspase 8/FADD interaction and their predicted docking energies are depicted: (b) F122 located on α2 helix of procaspase 8 DED2 is accommodated into a hydrophobic groove formed between α1 and α4 helices of FADD DED; (c) F25 located on α2 helix of FADD DED is accommodated into a hydrophobic groove formed between α1 and α4 helices of procaspase 8 DED1. (d) Western blot analysis of GST pull-down assay using FADD DED as bait and wild-type and mutant Flag-procaspase 8 constructs as prey. (e) Western blot analysis of a GST pull-down competition experiment, in which binding of Flag-tagged wild-type procaspase 8 and Flag-tagged wild-type FLIP(S) to the FADD DED was assessed in the presence or absence of the other protein. Procaspase 8 and FLIP(S) inputs were equalized prior to incubation with GST-FADD, and analysis of the first washes indicates that the pull downs were carried out with an excess of both Flag-tagged proteins. Figure 5: Molecular modelling and mutagenesis identify the predominant orientation for the procaspase 8–FADD interaction. ( a ) Homology model of human procaspase 8 DED1 and DED2 (light and dark magenta) superimposed on vFLIP X-ray protein (PDB id 2BBR; light green and green) and α3 region of FADD NMR-solved structure (PDB id 2GF5; dark green). The procaspase 8 DED1/2-MC159 identity is 29%; the r.m.s.d. calculated on Cα atoms is 1.03 Å. Two possible orientations of the procaspase 8/FADD interaction and their predicted docking energies are depicted: ( b ) F122 located on α2 helix of procaspase 8 DED2 is accommodated into a hydrophobic groove formed between α1 and α4 helices of FADD DED; ( c ) F25 located on α2 helix of FADD DED is accommodated into a hydrophobic groove formed between α1 and α4 helices of procaspase 8 DED1. ( d ) Western blot analysis of GST pull-down assay using FADD DED as bait and wild-type and mutant Flag-procaspase 8 constructs as prey. ( e ) Western blot analysis of a GST pull-down competition experiment, in which binding of Flag-tagged wild-type procaspase 8 and Flag-tagged wild-type FLIP(S) to the FADD DED was assessed in the presence or absence of the other protein. Procaspase 8 and FLIP(S) inputs were equalized prior to incubation with GST-FADD, and analysis of the first washes indicates that the pull downs were carried out with an excess of both Flag-tagged proteins. Full size image To assess the modelling predictions, we generated procaspase 8 F122A and Y8G single mutants and a F122A/Y8G double mutant. Consistent with the modelling predictions, the Y8G, but not the F122A mutant, exhibited significantly reduced binding to the FADD DED, while binding of the double mutant was further reduced ( Fig. 5d ). These results indicate that the predominant mode of interaction for procaspase 8 and FADD is the one depicted in Fig. 5c . Moreover, these results and those presented in Figs 2 , 3 , 4 suggest that FLIP and procaspase 8 do not compete with one another for binding to FADD in the manner previously thought, as each preferentially binds a different surface of the FADD DED. This was supported by pull-down studies in which we found that similar amounts of FLIP(S) and procaspase 8 interact with recombinant FADD regardless of the presence or absence of the other protein ( Fig. 5e ). In DISC IP assays, similar results were obtained, with the F122A mutant more efficiently recruited than Y8G ( Fig. 6a ). Importantly however, unlike the wild-type protein, DISC-recruited F122A mutant procaspase 8 was not significantly processed into p41 or p24 fragments, the latter fragment representing the N-terminal DED1/DED2 pro-domain detectable with the anti-FLAG antibody. Furthermore, neither the F122A nor the Y8G mutant forms of procaspase 8 could activate executioner caspases 3/7 in caspase 8 null Jurkat cells treated with TRAIL ( Fig. 6b ) nor initiate TRAIL-induced apoptosis in procaspase 8-depleted HCT116 cells ( Fig. 6c ). 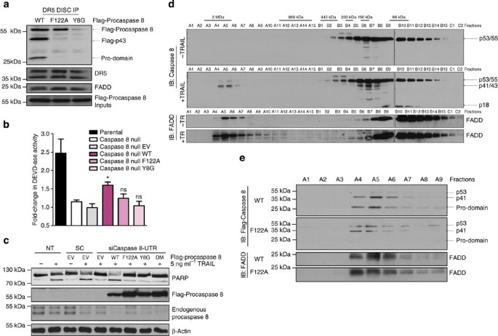Figure 6: Functional analyses of F122A and Y8G mutant procaspase 8. (a) Western blot analysis of DR5 DISC IP carried out in HCT116 cells expressing wild-type and mutant Flag-procaspase 8. Cells were transfected for 24 h prior to treatment. The DR5 DISC was captured 1 h after addition of anti-DR5-conjugated beads to cells. Co-immunoprecipitation of Flag-tagged procaspase 8 and FADD was assessed and pull down of DR5 confirmed. (b) Assessment of caspase 3/7-like DEVD-ase activity in parental and caspase 8 null Jurkat cells treated with 50 ng ml−1TRAIL for 6 h. The caspase 8 null cells were transfected with empty vector (EV) and wild-type (WT), F122A and Y8G mutant procaspase 8 as indicated. Mean values and s.d. are shown (n=3); *denotesP<0.05 compared with EV control as determined byt-test. (c) Assessment of apoptosis induced by rTRAIL in HCT116 cells overexpressing wild-type and mutant Flag-procaspase 8. Endogenous procaspase was downregulated by transfection with 20 nM of a 3′ UTR-targeted siRNA. Twenty-four hours following siRNA transfection, cells were transiently transfected with each construct for a further 24 h prior to treatment with 5 ng ml−1rTRAIL for 12 h. Apoptosis was assessed by PARP cleavage. (d) Western blot analysis of FADD and caspase 8 expression in HCT116 cells treated with 20 ng ml−1TRAIL for 3 h. Following treatment, cell lysates were prepared and passed through a size exclusion column. Fractions of different MW were collected as indicated by trace obtained from known MW standards. The results indicate that p53/55-procaspase 8 is processed to p41/43-caspase 8 in high-MW fractions following TRAIL treatment, with p18-caspase 8 appearing in the lower MW fractions. FADD was present in high-MW fractions in untreated cells, and its presence in the high MW fractions increased following TRAIL treatment. (e) Western blot analysis of size exclusion chromatography experiments in which HCT116 cells transfected with Flag-tagged wild-type (WT) or F122A mutant procaspase 8 were treated with 20 ng ml−1rTRAIL for 3 h prior to cell lysis and separation of low and high MW complexes using a size exclusion column. The expression of Flag-tagged procaspase 8 proteins and endogenous FADD were assessed by western blotting. Only the high-MW fractions are presented. Figure 6: Functional analyses of F122A and Y8G mutant procaspase 8. ( a ) Western blot analysis of DR5 DISC IP carried out in HCT116 cells expressing wild-type and mutant Flag-procaspase 8. Cells were transfected for 24 h prior to treatment. The DR5 DISC was captured 1 h after addition of anti-DR5-conjugated beads to cells. Co-immunoprecipitation of Flag-tagged procaspase 8 and FADD was assessed and pull down of DR5 confirmed. ( b ) Assessment of caspase 3/7-like DEVD-ase activity in parental and caspase 8 null Jurkat cells treated with 50 ng ml −1 TRAIL for 6 h. The caspase 8 null cells were transfected with empty vector (EV) and wild-type (WT), F122A and Y8G mutant procaspase 8 as indicated. Mean values and s.d. are shown ( n =3); *denotes P <0.05 compared with EV control as determined by t -test. ( c ) Assessment of apoptosis induced by rTRAIL in HCT116 cells overexpressing wild-type and mutant Flag-procaspase 8. Endogenous procaspase was downregulated by transfection with 20 nM of a 3′ UTR-targeted siRNA. Twenty-four hours following siRNA transfection, cells were transiently transfected with each construct for a further 24 h prior to treatment with 5 ng ml −1 rTRAIL for 12 h. Apoptosis was assessed by PARP cleavage. ( d ) Western blot analysis of FADD and caspase 8 expression in HCT116 cells treated with 20 ng ml −1 TRAIL for 3 h. Following treatment, cell lysates were prepared and passed through a size exclusion column. Fractions of different MW were collected as indicated by trace obtained from known MW standards. The results indicate that p53/55-procaspase 8 is processed to p41/43-caspase 8 in high-MW fractions following TRAIL treatment, with p18-caspase 8 appearing in the lower MW fractions. FADD was present in high-MW fractions in untreated cells, and its presence in the high MW fractions increased following TRAIL treatment. ( e ) Western blot analysis of size exclusion chromatography experiments in which HCT116 cells transfected with Flag-tagged wild-type (WT) or F122A mutant procaspase 8 were treated with 20 ng ml −1 rTRAIL for 3 h prior to cell lysis and separation of low and high MW complexes using a size exclusion column. The expression of Flag-tagged procaspase 8 proteins and endogenous FADD were assessed by western blotting. Only the high-MW fractions are presented. Full size image Using size exclusion chromatography, we found that TRAIL treatment resulted in recruitment of procaspase 8 into high-molecular weight (MW) complexes of ~2 MDa, where it was detected predominantly as its partially processed p41/43 forms ( Fig. 6d ). p18-caspase 8 was detected in lower MW fractions (~60 kDa) from TRAIL-treated cells consistent with the dissociation of the active p10/p18 hetero-tetramer from the DISC. Interestingly, FADD was detectable in the high-MW fractions prior to treatment, indicating that a proportion of FADD is constitutively associated with macro-molecular complexes ( Fig. 6d ); treatment with TRAIL significantly increased the proportion of FADD in these high-MW complexes. Although F122A procaspase 8 was recruited into these high-MW fractions following TRAIL treatment, it was inefficiently processed into the p41 fragment and no pro-domain fragment was detected ( Fig. 6e ). In contrast, FLAG-tagged wild-type procaspase 8 was detected exclusively as p41 and pro-domain fragments, indicative of highly efficient processing. Collectively, the results presented in Figs 5 , 6 indicate that procaspase 8 predominantly uses Y8 on the α1/α4 surface of DED1 to interact with FADD at the DISC and that F122 in the α2/α5 DED2 binding interface is necessary for procaspase 8 to undergo full processing and activation at the DISC. A two-step model of DED protein assembly at the DISC To account for the above results, we propose a model of DISC assembly, in which FADD binding to DR5 via its DD releases both faces of the FADD DED to become available for forming protein–protein interactions ( Fig. 7a ). Then, due to their relative affinities for the two faces of the FADD DED, FLIP preferentially binds to the α1/α4 surface and procaspase 8 to the α2/α5 surface to form a tripartite FLIP–FADD–procaspase 8 DED complex ( Fig. 7a , step 1). Subsequently, these tripartite complexes interact with one another via the DED surfaces in FLIP and procaspase 8 that are still available for forming protein–protein interactions (the α1/α4 surface of FLIP and the α2/α5 surface of procaspase 8; Fig. 7a , step 2). When FLIP(L) is recruited to FADD α1/α4, interaction with procaspase 8 in an adjacent DED trimer would allow interaction between the caspase-like domain of FLIP(L) and the caspase domain of caspase 8, leading to formation of the catalytically active but membrane-restricted and apoptosis-incompetent p43-FLIP(L)-p41/43-caspase 8 enzyme [32] . When FLIP(S) is recruited to FADD α1/α4, its lack of caspase-like domain would mean that its interaction with procaspase 8 in an adjacent trimer would not lead to the conformational changes in the catalytic domain necessary to activate the procaspase. Thus, recruitment of either FLIP splice form to FADD α1/α4 blocks processing of procaspase 8 into an apoptosis-inducing caspase. However, when FLIP levels become depleted, the more highly expressed procaspase 8 starts to be recruited to the α1/α4 surface of the FADD DED as well as its more favoured α2/α5 surface, with the result that interactions between adjacent trimers can now lead to the formation of procaspase 8 homodimers and processing into the apoptosis-competent caspase. Such a model of DISC assembly proposes that ultimately procaspase 8-FLIP hetero-dimerization or procaspase 8 homodimerization occurs as depicted in Fig. 7b , with two flanking FADD DEDs. 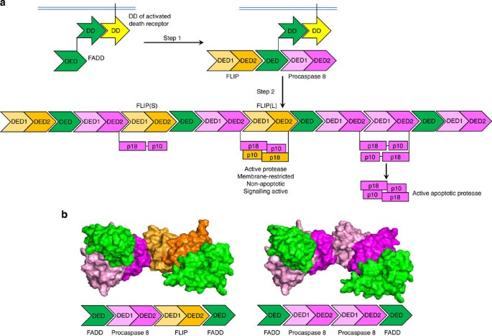Figure 7: A novel two-step DISC model. (a) Proposed model of DISC assembly: following binding of TRAIL to DR5, the DD of the death receptor become available for interaction with DD of FADD. Once bound via its DD to a DR, the DED of FADD (green chevrons) can form protein–protein interactions with the DEDs of procaspase 8 (purple chevrons) and FLIP (orange chevrons) (step 1). Owing to their relative binding affinities, FLIP is primarily recruited to the α1/α4 face of FADD and procaspase 8 to the α2/α5 surface to form intermediate tripartite complexes. Individual tripartite complexes then interact with one another via interactions between the α1/α4 face of FLIP and the α2/α5 surface of procaspase 8 (step 2). When FLIP(S) is recruited to the α1/α4 surface of the FADD DED, procaspase 8 remains unprocessed; however, when FLIP(L) is recruited, interaction with procaspase 8 in an adjacent DED trimer would allow interaction between the caspase-like domain of FLIP(L) and the caspase domain of caspase 8, leading to formation of the apoptosis-incompetent, membrane-restricted but catalytically active p43-FLIP(L)-p41/43-caspase 8 enzyme that can act on local substrates such as RIPK1. When FLIP levels become depleted (for example, at high levels of receptor stimulation), procaspase 8 is recruited more frequently to the α1/α4 surface of the FADD DED as well as the α2/α5 surface, interactions between adjacent trimers can now lead to the formation of procaspase 8 homodimers and processing into the apoptosis-competent caspase. (b) Molecular modelling of the proposed FADD-procaspase 8-FLIP/procaspase 8-FADD interactions at the DISC. Figure 7: A novel two-step DISC model. ( a ) Proposed model of DISC assembly: following binding of TRAIL to DR5, the DD of the death receptor become available for interaction with DD of FADD. Once bound via its DD to a DR, the DED of FADD (green chevrons) can form protein–protein interactions with the DEDs of procaspase 8 (purple chevrons) and FLIP (orange chevrons) (step 1). Owing to their relative binding affinities, FLIP is primarily recruited to the α1/α4 face of FADD and procaspase 8 to the α2/α5 surface to form intermediate tripartite complexes. Individual tripartite complexes then interact with one another via interactions between the α1/α4 face of FLIP and the α2/α5 surface of procaspase 8 (step 2). When FLIP(S) is recruited to the α1/α4 surface of the FADD DED, procaspase 8 remains unprocessed; however, when FLIP(L) is recruited, interaction with procaspase 8 in an adjacent DED trimer would allow interaction between the caspase-like domain of FLIP(L) and the caspase domain of caspase 8, leading to formation of the apoptosis-incompetent, membrane-restricted but catalytically active p43-FLIP(L)-p41/43-caspase 8 enzyme that can act on local substrates such as RIPK1. When FLIP levels become depleted (for example, at high levels of receptor stimulation), procaspase 8 is recruited more frequently to the α1/α4 surface of the FADD DED as well as the α2/α5 surface, interactions between adjacent trimers can now lead to the formation of procaspase 8 homodimers and processing into the apoptosis-competent caspase. ( b ) Molecular modelling of the proposed FADD-procaspase 8-FLIP/procaspase 8-FADD interactions at the DISC. Full size image This model is consistent with the DISC stoichiometry we observed of two FLIP/caspase 8 molecules for every FADD molecule ( Fig. 1 ). The model also suggests that the interaction between procaspase 8 and FLIP following assembly of the initial tripartite complex is mediated via interactions between DED2 of procaspase 8 and DED1 of FLIP. Molecular docking studies suggested that procaspase 8 F122 would be critical for mediating this interaction ( Fig. 8a ) and that between two molecules of procaspase 8 ( Fig. 8b ). To assess this, we performed pull-down assays using His-tagged FLIP or caspase 8 DED1/2 and Flag-tagged wild-type and mutant versions of full-length and the DED-only region of procaspase 8. In contrast to its interaction with FADD ( Fig. 5 ), it was found that procaspase 8 is highly dependent on F122 rather than Y8 to interact with itself and FLIP ( Fig. 8c ). These results are consistent with those presented in Fig. 6 in which F122A procaspase 8 is recruited to the DISC but is inefficiently processed and cannot trigger apoptosis induction: procaspase 8 processing occurs following homodimerization with another molecule of procaspase 8 (which generates p41/43 and pro-domain fragments and the active p10/p18 heterotetrameric enzyme in two sequential cleavage events) or heterodimerization with FLIP(L) (which generates p41/43 fragments via a single-cleavage event). 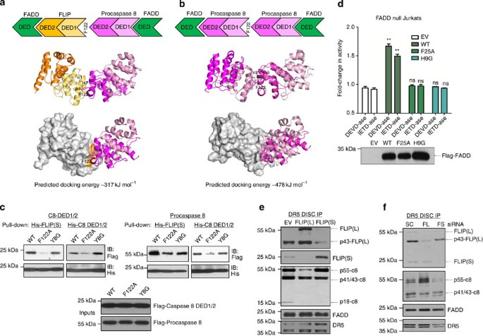Figure 8: Testing predictions of the two-step DISC model. Molecular models of the inter-molecular DED interactions between FLIP and procaspase 8 (a) and two procaspase 8 molecules (b) that are predicted to occur in the proposed two-step model of DISC assembly. In these models, F122 located on α2 helix of procaspase 8 DED2 is accommodated into a hydrophobic groove formed between α1 and α4 helices of the FLIP or procaspase 8 DED1. (c) Western blot analysis of pull-down experiments using His-tagged FLIP or procaspase 8 DED1/2 as ‘bait’ and Flag-tagged wild-type and mutant full-length and DED-only procaspase 8 as ‘prey’. (d) Assessment of caspase activation induced by rTRAIL in FADD null Jurkat cells transfected with wild-type or mutant Flag-tagged FADD constructs. Twenty-four hours following transfection, cells were treated with 50 ng ml−1rTRAIL for 6 h prior to assessment of caspase 3/7-like (DEVD-ase) and caspase 8-like (IETD-ase) activity. Mean values and s.d. are shown (n=3); **P<0.01 compared with EV control as determined byt-test. (e) Western blot analysis of DR5 DISC IP carried out in Ren mesothelioma cells overexpressing FLIP(L) or FLIP(S). The DISC was captured 1 h after addition of anti-DR5-beads to cells. (f) Western blot analysis of DR5 DISC IP carried out in HCT116 colon cancer cells transfected with 10 nM control siRNA (SC), FLIP(L)-specific siRNA (FL), FLIP(S)-specific siRNA (FS) or dual FLIP(L)/(S)-targeted siRNA (FT). Cells were transfected for 24 h and co-treated with 10 μM z-VAD-fmk to prevent apoptosis induced by FLIP silencing (z-VAD-fmk does not inhibit processing of p53/55-procaspase 8 to p41/43-caspase 8, but does prevent further processing). The DR5 DISC was captured 1 h after addition of anti-DR5-Beads to cells. Figure 8: Testing predictions of the two-step DISC model. Molecular models of the inter-molecular DED interactions between FLIP and procaspase 8 ( a ) and two procaspase 8 molecules ( b ) that are predicted to occur in the proposed two-step model of DISC assembly. In these models, F122 located on α2 helix of procaspase 8 DED2 is accommodated into a hydrophobic groove formed between α1 and α4 helices of the FLIP or procaspase 8 DED1. ( c ) Western blot analysis of pull-down experiments using His-tagged FLIP or procaspase 8 DED1/2 as ‘bait’ and Flag-tagged wild-type and mutant full-length and DED-only procaspase 8 as ‘prey’. ( d ) Assessment of caspase activation induced by rTRAIL in FADD null Jurkat cells transfected with wild-type or mutant Flag-tagged FADD constructs. Twenty-four hours following transfection, cells were treated with 50 ng ml −1 rTRAIL for 6 h prior to assessment of caspase 3/7-like (DEVD-ase) and caspase 8-like (IETD-ase) activity. Mean values and s.d. are shown ( n =3); ** P <0.01 compared with EV control as determined by t -test. ( e ) Western blot analysis of DR5 DISC IP carried out in Ren mesothelioma cells overexpressing FLIP(L) or FLIP(S). The DISC was captured 1 h after addition of anti-DR5-beads to cells. ( f ) Western blot analysis of DR5 DISC IP carried out in HCT116 colon cancer cells transfected with 10 nM control siRNA (SC), FLIP(L)-specific siRNA (FL), FLIP(S)-specific siRNA (FS) or dual FLIP(L)/(S)-targeted siRNA (FT). Cells were transfected for 24 h and co-treated with 10 μM z-VAD-fmk to prevent apoptosis induced by FLIP silencing (z-VAD-fmk does not inhibit processing of p53/55-procaspase 8 to p41/43-caspase 8, but does prevent further processing). The DR5 DISC was captured 1 h after addition of anti-DR5-Beads to cells. Full size image The proposed two-step model also suggests that both binding surfaces of the FADD DED are required to form an apoptosis-competent DISC. To test this, we assessed the ability of FADD F25A and H9G mutants to activate TRAIL-induced apoptosis. Consistent with our model, wild-type FADD, but neither the F25A nor H9G mutant, was able to induce TRAIL-induced caspase 8 and caspase 3/7 activation when transiently transfected into FADD null Jurkat cells ( Fig. 8d ). In addition, due to its lower affinity for the FADD α2/α5 surface and low expression levels compared with procaspase 8 ( Fig. 1g ), our model would predict that only rarely or at supra-physiological expression levels are FLIP homodimers generated at the DISC; in the case of FLIP(L), the presence of such homodimers is revealed by the detection of unprocessed p55-FLIP(L) in the DISC IP obtained from Ren cells that highly overexpress FLIP(L) ( Fig. 8e ). Also, the model predicts that when FLIP(L) is the predominant form of FLIP recruited, caspase 8 will be detected predominantly in its p41/43 form, but when FLIP(S) is the predominant splice form, procaspase 8 will be detected predominantly in its unprocessed p53/55 form; indeed, this is exactly what is observed in cells in which each splice form is overexpressed ( Fig. 8e ) or selectively downregulated ( Fig. 8f ). It is essential that activation of initiator caspases such as caspase 8 is tightly regulated. In this study, we identified the predominant modes with which FADD interacts with procaspase 8 and its endogenous inhibitor FLIP at the DR5 DISC. In addition to the previously identified highly conserved phenylalanine (F) residue in DED α2 (ref. 31 ), we identified another conserved aromatic residue (H or Y) on α1 of FADD DED and DED1 of procaspase 8 that is also critical for DISC assembly. Indeed, we report for the first time that both the α1/α4 and α2/α5 surfaces of all three proteins are involved in regulating protein–protein interactions at the DISC and are necessary for the pro-apoptotic functions of FADD and procaspase 8. Overall, our results support a ‘two-step’ model of DISC assembly as depicted in Fig. 7a , in which binding of the FADD DD to DR5 releases its DED [24] ; then, due to their preferential binding affinities, FLIP binds the FADD DED α1/α4 surface and procaspase 8 binds the α2/α5 surface. In the second step, individual tripartite complexes interact with one another via reciprocal interactions between the α1/α4 surface of FLIP and the α2/α5 surface of procaspase 8, in which procaspase 8 F122 plays a key role. As levels of DISC stimulation increase, the levels of FLIP become depleted, and procaspase 8 is recruited more frequently to the FADD DED α1/α4 surface as well as the α2/α5 surface; this in turn leads to formation of procaspase 8 homodimers when neighbouring tripartite complexes interact (with F122 again important), enabling the dimerization of its caspase domains that is necessary to generate the active enzyme [32] . Our study also resolves the role of the conserved E-RxDL charged triad motifs of FLIP [30] , [33] , [34] , which maintain the structural topography and correct spatial orientations of α2/α5 and α1/α4 helices. Our proposed model is consistent with the preference for FADD to engage procaspase 8 via its α2/α5 surface and FLIP with its α1/α4 surface ( Figs 3 and 5 ). This model also explains the requirement for FLIP F114 for its interaction with FADD and DISC recruitment and how by only binding the α1/α4 surface of FADD, the FLIP H7G mutant can block TRAIL-induced apoptosis almost as efficiently as the wild-type protein ( Fig. 4 ). In addition, this model can explain why F122A procaspase 8 can interact with FADD and is recruited to the DISC, but does not get efficiently processed and cannot activate apoptosis ( Fig. 6 ): when bound to FADD via the α1/α4 surface of its first DED, F122A procaspase 8 does not efficiently engage another molecule of procaspase 8 via its second DED. Moreover, as Y8G procaspase 8 must predominantly use its α2/α5 surface to bind other DEDs, it has to compete directly with FLIP for binding to the α1/α4 surface of FADD; given the relative affinities of procaspase 8 and FLIP for this surface of FADD, this explains why recruitment of this mutant to the DISC is inefficient ( Fig. 6a ). Recently proposed models of the interactions between the DDs of FADD and the DDs of Fas predict that either four or five FADD DEDs are positioned around the perimeter of a core oligomeric complex that is held together by interactions between the DDs of Fas and FADD [15] , [24] , [35] . It is possible that the FADD DEDs in these complexes are spatially arranged to promote interactions between procaspase 8 and FLIP molecules that are recruited to adjacent FADD DEDs. Interestingly, our modelling suggests that FADD-procaspase 8-FLIP/procaspase 8-FADD DED complexes possess curvature ( Fig. 7b ) that could facilitate bridging interactions between adjacent FADD DEDs in such higher-order structures. Our DED assembly model is also consistent with the highly oligomeric nature of both proposed DD assembly models and would predict a DISC of MW similar to that observed by us ( Fig. 6d ) and others. Although our two-step DISC DED assembly model differs with the procaspase 8 chain model proposed by Dickens et al. [25] and Schleich et al. [26] , our results are similar to the ~2:1–3:1 procaspase 8:FADD ratios obtained in several experiments in these studies using quantitative mass spectrometry. However, our results differ with the quantitative western analyses of Schleich et al. [26] A potential explanation for this difference is the use of GST-FADD as a standard [36] , as we found that GST-FADD and GST-FLIP proteins gave signals ~5–10 times higher than equimolar amounts of the untagged proteins ( Supplementary Fig. S5 ); although the reasons for this are unclear, using GST-FADD and GST-FLIP proteins as standards could lead to a significant underestimation of the amount FADD and FLIP at the DISC. Work from our group and others implicate FLIP as a potential anticancer therapeutic target [11] . Conventional homotypic DED interaction models for DISC assembly suggest that therapeutically targeting FLIP recruitment to the DISC may not be feasible without disrupting procaspase 8 recruitment. The data presented in this study challenge this notion as they indicate that there are important differences between FLIP and procaspase 8 in terms of their binding affinities and preferred modes of interaction with the α1/α4 and α2/α5 surfaces of FADD that could be therapeutically exploited to promote TRAIL agonist-induced apoptosis. These results also have broader biological and clinical implications as they reveal a novel model of DED protein assembly that may also explain how the enzymatic activities of the Fas DISC, TNFR1 Complex II and Ripoptosome are regulated. Cell culture and transfection HCT116 cells, which were a kind gift from Professor B Vogelstein (Johns Hopkins University School of Medicine, Baltimore), were cultured in McCoy’s medium supplemented with 10% FCS (Invitrogen, Paisley UK). Jurkat, A549 and H460 cells were obtained from ATCC (Teddington, UK). Jurkat cells were maintained in RPMI1640 supplemented with 10% FCS; A549 and H460 cells were maintained in DMEM supplemented with 10% FCS. REN cells stably over-expressing FLIP L , FLIP S or an empty vector (EV) control were generated as previously described [28] and maintained in F-12 (Ham) medium supplemented with 10% FCS. All cell lines were maintained in 5% CO 2 at 37 °C and regularly screened for the presence of mycoplasma using the MycoAlert Mycoplasma Detection Kit (Lonza, Basel, Switzerland). Cell lines were validated by STR profiling. DNA transfection of HCT116 cells was carried out using Genejuice reagent (Invitrogen). DNA transfection of Jurkat cells was carried out using Xtreme gene-HP reagent (Roche). The non-silencing control (SC) siRNA, FLIP and caspase 8 siRNAs were obtained from Dharmacon (Chicago, IL). The siRNA sequences were as follows: FLIP(L)/(S): 5′-AAGCAGUCUGUUCAAGGAGCA-3′; FLIP(L): 5′-AAGGAACAGCUUGGCGCUCAA-3′; FLIP(S): 5′-AACAUGGAACUGCCUCUACUU-3′; caspase 8 UTR#1: 5′-UAGCUGGUGGCAAUAAAUA-3′; caspase 8 UTR#2: 5′-UUAGCUGGUGGCAAUAAAU-3′; and control sequence: 5′-AAUUCUCCGAACGUGUCACGU-3′. siRNA transfections were carried out using OligofectAMINE (Invitrogen). All transfections were carried out according to the manufacturers’ instructions. Homology models of human FLIP and procaspase 8 The primary sequences of human FLIP (sp O15519) and procaspase 8 (sp Q14790) were taken from UniProt database. Homology models of the DEDs of human FLIP and procaspase 8 were built with MODELLER9 version 8 (ref. 37 ) using the X-ray structure of viral FLIP MC159 (PDB id 2BRR) as a template (ref. 29 ). A classification of DED-containing proteins based on the high diversity of the α3 region helped us to refine the models [38] . In this classification, DED of FADD, DED2 of FLIP, and both DEDs of procaspase 8 belong to the same class (class I) and contain basic residues (K or R). As observed in the NMR-solved structure of FADD (PDB id 2GF5) [39] , these residues form a short α-helix (α3 helix). In contrast, both DEDs of viral FLIP MC159 and the DED1 of human FLIP belong to a different DED class (II) because they do not contain these basic residues. In the viral FLIP crystal structure, the α3 region is a loop. Thus, we refined the α3 region of FLIP DED2 and both procaspase 8 DEDs using the α3 helix of FADD DED as template. The three-dimensional quality of the structures was validated using ProSa2003 programme ( http://www.came.sbg.ac.at/prosa_details.php ) [40] . The models showing the best scores as judged by consensus predictions carried out by MODELLER objective function and ProSa2003 were chosen. PDB coordinate files are available from the corresponding author subject to a confidentiality agreement. Protein–protein docking analyses The docking of FLIP-FADD, procaspase 8-FADD, procaspase 8-procaspase 8, FLIP-FLIP and procaspase 8-FLIP DEDs was performed with Hex software [41] . Firstly, manual positioning of the two possible orientations for FLIP-FADD and procaspase 8-FADD was obtained, and these were used as reference complexes in Hex. The HEX docking algorithm employs molecular shape comparison using spherical harmonics and polar Fourier correlations. The initial steric scan was set at N =16 followed by a final search at N =25. This discards orientations where a steric clash occurs during the rigid body-docking procedure that employs shape (steric) and electrostatic correlation. The twist range angle was set at 360° with a step size of 5.5°. The docking calculations were performed using 12 inter-molecular separations in steps of 7.5 Å. The solutions with the lowest root mean square deviation (r.m.s.d.) with respect to the reference complex was chosen. Antibodies Anti-FADD (A66-2, Pharmingen) (1:2,000), anti-PARP (C2-10, eBioscience) (1:5,000), anti-FLAG-HRP (M2, Sigma) (1:2,000), anti-FLIP (NF6, Alexis) (1:1,000), anti-caspase 8 (12F5, Alexis) (1:5,000), anti-GST-HRP (DG122-2A7, Merck Millipore) (1:10,000), anti-caspase-10 (4C1, MBL) (1:1,000) and anti-DR5 (catalogue number 3696, Cell Signalling) (1:2,000) antibodies were used in western blot analyses. Caspase-8 p18 antibody (c20, Santa Cruz) (5 μg per sample) was used for immunoprecipitation. Expression constructs Flag-tagged FLIP L , FLIP S , FADD and procaspase 8 expression constructs were generated in the pCMV-3Tag-6 vector (Agilent Technologies). GST-tagged FLIP S and FADD expression constructs were generated in the pGEX-6P-3 vector (GE Healthcare). Mutagenesis was carried out using the KOD Extreme polymerase (Novagen), with the template plasmid digested using DpnI (New England Biolabs). DR5 DISC assay AMG655 (Conatumumab) was a kind gift from Amgen. This fully humanized antibody, which recognizes the extracellular region of DR5, was conjugated to Dynabeads using the antibody coupling kit from Invitrogen as per the manufacturer’s instructions. For the DR5 DISC assay, 30 μl of Dynabeads coated with 5 μg of AMG655 was added to 2 × 10 6 cells and incubated for 1 h. The cells were then lysed in DISC buffer (0.2% NP-40, 20 mM Tris-HCL (pH 7.4), 150 mM NaCl and 10% glycerol). The AMG655-coated Dynabeads were collected and washed 5 times in DISC buffer prior to resuspension in Laemmli buffer and analysis by western blotting. Supernatants and inputs were also collected and analysed by western blotting. Immunoprecipitation (IP) reactions Protein lysates were prepared using CHAPS buffer (10 mM HEPES, 150 mM NaCl, 1% CHAPS, pH 7.4). Lysates (2 mg) were pre-cleared overnight with sheep anti-rabbit IgG Dynabeads (Invitrogen). Anti-caspase 8 antibody (2 μg) was conjugated with sheep anti-rabbit IgG Dynabeads for at least 1 h and then washed prior to incubation with pre-cleared lysates for at least 4 h. After several washes, Dynabeads were resuspended in Laemmli loading buffer and heated at 95 °C for 5 min prior to immunoblot analysis. Caspase activity assay Caspase 8 or caspase 3/7-GLO reagents (25 μl) (Promega) were incubated with 1–10 μg of protein lysate diluted in cell culture medium in a total volume of 50 μl for 1–2 h at room temperature. Luciferase activity was then determined using a luminometer. Recombinant protein purification and GST pull downs GST, GST-tagged FLIP S and GST-tagged FADD were expressed in IPTG-stimulated BL21 bacteria. Bacterial cell lysates were purified using Glutathione-Sepharose beads (GE Healthcare BioSciences AB) and dialysed using Slide-A-Lyzer Dialysis Cassettes (Thermo Scientific). For pull downs, GST-tagged proteins (5 μg) were conjugated to Glutathione–Sepharose beads and incubated with pre-cleared protein lysates (500 μg) for 2 h at 4 °C with constant mixing. Beads were washed several times in RIPA buffer and resuspended in Laemmli buffer prior to western blot analysis. For quantitative western blotting and His-pull-downs, a His-tagged FLIP S expression construct was generated in the pET45(b) vector and recombinant protein expressed and purified from IPTG-stimulated BL21 bacteria using Ni-NTA agarose beads (Qiagen). A His-tagged caspase 8 DED-only construct was similarly generated and expressed. His-pull-down experiments were conducted using Ni-NTA agarose beads in a manner similar to GST-pull down described above. For quantitative western blotting of FADD, the GST-tag was cleaved from the GST-FADD fusion protein using PreScission Protease (GE Helathcare). For quantitative western blotting of caspase 8 recombinant p18-caspase 8 was purchased from Sigma. The concentrations of all the recombinant proteins used in quantitative western blotting applications were quantified using the micro-BCA system (Pierce). Quantitative DISC (Q-DISC) and western blot analyses For the Q-DISC, cells seeded the previous day at 5 × 10 6 were exposed to crosslinked anti-DR5 antibody, and 20% of each DISC IP was analysed for FLIP, FADD and caspase 8 recruitment. For quantifying the number of protein molecules per cell, lysates from 100,000 cells were prepared. Recombinant proteins for FLIP (His-tagged), FADD (untagged) and caspase 8 (p18, Sigma) were used as standards. Anti-FADD (Pharmingen), anti-FLIP (NF6, Alexis) and anti-caspase 8 (12F5, Alexis) antibodies were used in conjunction with a goat anti-mouse IRDye 800CW secondary antibody, and bands were detected and quantified using the Odyssey Infrared Imaging System (LI-COR Biosciences, UK). For FLIP, the amounts of FLIP(S) and FLIP(L) were added together, while for caspase 8, the bands corresponding to p53/p55 and p41/43 caspase 8 were added. Uncropped western blots are presented in Supplementary Fig. 6 . Size exclusion chromatography Cell lysates were prepared and subjected to size exclusion chromatography using the Superose 6 10/300 GL column and AKTA purifier (both GE Healthcare) as previously described [8] . Fractions of different MW were collected and subjected to western blotting analyses. The MW of fractions was assessed by comparison with a trace obtained from known MW standards (Sigma). Statistical analysis Experimental results were compared using a two-tailed Student’s t -test; * P <0.05, ** P <0.01 and *** P <0.001. All experiments were replicated at least two times and in most cases, more than three times. How to cite this article: Majkut, J. et al. Differential affinity of FLIP and procaspase 8 for FADD’s DED binding surfaces regulates DISC assembly. Nat. Commun. 5:3350 doi: 10.1038/ncomms4350 (2014).